All-solution processed polymer light-emitting diode displays Adopting the emerging technology of printed electronics in manufacturing novel ultrathin flat panel displays attracts both academic and industrial interests because of the challenge in the device physics and the potential of reducing production costs. Here we produce all-solution processed polymer light-emitting diode displays by solution-depositing the cathode and utilizing a multifunctional buffer layer between the cathode and the organic layers. The use of ink-jetted conducting nanoparticles as the cathode yields high-resolution cathode patterns without any mechanical stress on the organic layers. The buffer layer, which offers the functions of solvent-proof electron injection and proper affinity, is fabricated by mixing the water/alcohol-soluble polymer and a curable epoxy adhesive. Our 1.5-inch polymer light-emitting diode displays are fabricated without any dead pixels or dead lines. The all-solution process eliminates the need for high vacuum for thermal evaporation of the cathode, which paves the way to industrial roll-to-roll manufacturing of flat panel displays. In 1987, Kodak’s Tang and Vanslyke [1] reported on the first low-voltage, high-efficiency, thin-solid-film small-molecule organic light-emitting diode (OLED). The basic device structure consisted of a bilayer structure, in which the hole-transport layer and the emission layer were sandwiched between two charge injection contact electrodes. To date, almost all the active layers in small-molecule OLEDs, as well as the cathodes, are deposited via high-vacuum evaporation, leading to high production cost, low yield and limited device size [2] , [3] . In 1990, Friend et al . introduced a conjugated polymer poly(phenylene-vinylene) (PPV) as the light-emitting material, and fabricated the first polymer light-emitting diode (PLED) [4] . The next year, Braun and Heeger further improved the insoluble polymer PPV to the soluble polymer poly(2-methoxy-5-(2′-ethyl-hexoxy)-1,4-phenylene-vinylene) (MEH-PPV; Fig. 1 ) [5] , which introduced the solution process to OLED/PLED manufacturing. Compared with vacuum deposition, the solution process is simpler and less expensive. Various solution processes have been successfully developed, such as spin-coating [3] , inkjet printing [6] , screen printing [7] , dye diffusion [8] , micro-molding in capillary [9] , micro-contact printing [10] , photolithographic process [11] and dip-coating [12] . The solution process is typically performed at low or room temperature, enabling a device to be fabricated onto a flexible, organic substrate [13] . 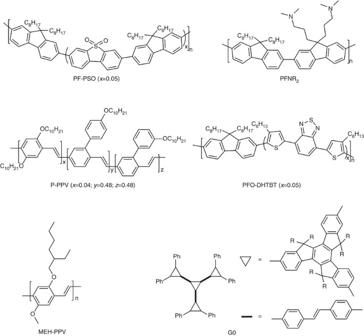Figure 1: Molecular structures of the materials used in the experiments. MEH-PPV and PFO-DHTBT (poly[4,7-di(4-hexyl-2-thienyl)-2,1,3-benzothiadiazole-co-(9,9-dioctyl)-2,7-fluorene]) are red emitters. P-PPV is a green emitter. The dentrimer G0 and PF-FSO are blue emitters. PFNR2is an electron-injection material. Figure 1: Molecular structures of the materials used in the experiments. MEH-PPV and PFO-DHTBT (poly[4,7-di(4-hexyl-2-thienyl)-2,1,3-benzothiadiazole-co-(9,9-dioctyl)-2,7-fluorene]) are red emitters. P-PPV is a green emitter. The dentrimer G0 and PF-FSO are blue emitters. PFNR 2 is an electron-injection material. Full size image Although the organic functional layers in PLEDs are solution-processed, the cathodes are still deposited via thermal evaporation in a high-vacuum chamber. The commonly used cathode materials, that is, low work function metals [5] , [14] , alkaline halides and alkali-earth halides [15] , [16] , cannot be stably dissolved or dispersed in solvents. To screen-print silver paste as the cathode, Add-Vision Inc. (now part of Sumitomo Chemical) adopted the light-emitting electrochemical cell technology to fabricate a fully solution-processed display [17] , [18] . However, the screen-printing process for cathode deposition limits the display to low resolution, and the light-emitting electrochemical cell device structure has an intrinsically slow response time that is not suitable for video applications. Recently, our laboratory synthesized a novel water/alcohol-soluble conjugated polyfluorene polyelectrolyte poly[(9,9-bis(3'-(N,N-dimethylamino)propyl)-2,7-fluorene)-alt-2,7-(9,9-dioctylfluorene)] (PFNR 2 ; Fig. 1 ) [19] , to serve as the highly efficient electron-injection layer (EIL) between high work function metals and light-emitting polymers [20] , [21] . The introduction of water/alcohol-soluble EIL into PLEDs maintains the LED characteristics [22] , [23] , which makes it possible to fabricate PLEDs using an all-solution process with high resolution and fast response time. Red-, green- and blue-emission PLED single devices with 3 × 3 cm 2 active areas were fabricated without any vacuum process using blade-coating silver paste as the cathode on top of PFNR 2 EIL in nitrogen [24] . Unfortunately, the solvents (dispersants) in the conducting pastes easily permeated into the underlying organic layers and damaged the layers, which reduced the device performance and stability. Thus, the solvents must be controlled to a very low level, thereby limiting the selection of printing methods and restricting the pattern quality. Moreover, the micro-sized metal particles easily pierce the organic layers, which are fragile and thin (with total thicknesses of less than 150 nm). Unlike in PLED single devices, the cathodes need to be patterned in flat panel displays. A high-resolution display requires fine cathode lines with high electric conductivity along the lines and good electric isolation between adjacent lines. Neither blade-coating nor screen-printing nor the conducting paste developed for PLED single devices meets such demands. The inkjet process is a good candidate for printing super-fine patterns [25] , [26] . To apply the inkjet process in cathode printing, the printable cathode materials must contain enough solvents, that is, dilute ‘inks’, to attain the viscosity and surface tension required by the inkjet printer. As we mentioned earlier, however, extra solvents will penetrate into the organic functional layers, which causes a large current leakage to develop. The leakage current in PLED displays will cause serious dead line defects. To overcome this issue, a buffer layer (BL) between the organic layers and the printed cathode must be introduced to block the attack from the solvent of the cathode ink while also providing efficient electron injection from the cathode. In this work, we blend an epoxy adhesive, ELC 2500CL from Electro-Lite Corp., and PFNR 2 at a weight ratio of 10:2 to fabricate a 50 nm BL on top of an emission layer. The epoxy, after curing, crosslinks to form a stable three-dimensional copolymer net that is impenetrable by common solvents. Doping the epoxy with the water-soluble conjugated polymer PFNR 2 provides the film formability and the necessary electron injection and adjusts the surface energy to offer good affinity with the printed cathode. The BL ensures the success of defect-free, good performance and high-resolution PLED displays produced using an all-solution process. By combining the multifunctional BL with ink-jetting conducting nanoparticles as the cathode, 1.5-inch diagonal red, green, blue monochrome and full-colour PLED displays with a content format of 96 × 3 × 64 pixels are successfully fabricated without any dead pixels or dead lines. Removing the vacuum and high-temperature processes in PLED display fabrication significantly reduces the production cost, which provides PLED technology with an additional incentive to manufacture using the industrial roll-to-roll process. Single device To demonstrate the functions of the BL in the all-solution process, a PLED single device with the structure presented in Fig. 2a was fabricated. On top of the transparent substrate ITO glass, a 50-nm thick poly(3,4-ethylenedioxythiophene):poly(styrenesulfonate) (PEDOT:PSS) hole-injection layer, a 80-nm thick poly[2-(4-(3′,7′-dimethyloctyloxy)-phenyl)- p -phenylene-vinylene] (P-PPV; Fig. 1 ) [27] emission layer and a 50-nm thick epoxy:PFNR 2 BL were spin-coated sequentially. A detailed description of the device fabrication is provided in the Methods. The optimization of the layer thickness and the characterization of the curing condition are described in Supplementary Tables S1 and S2 . After an ultraviolet and low-temperature annealing process to cure the BL, nano silver ink (DGP 40LT-15C from ANP Ltd., solid content 35%) was deposited as the cathode in air at room temperature using an inkjet printer (DMP 2831 from FUJIFILM Dimatix Inc.) followed by 30 min annealing at 140 °C. Transmission electron microscopy (TEM) images of the silver nanoparticles are presented in Fig. 2b . Before curing, the mean particle size was 44.2 nm, and the particle shape was polyhedron. After annealing, the silver nanoparticles became sphere-shaped and formed a solid and continuous film with a thickness of approximately 1 μm and a resistivity of approximately 3.6 × 10 −7 Ωm. 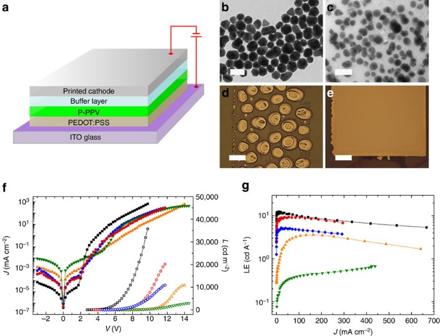Figure 2: Single PLED device structure and performance with various EIL or BL and cathode combinations. (a) Device structure of the all-solution processed PLED single device with the printed nanoparticle cathode. (b) TEM image of the silver nanoparticles before curing. The nanoparticles have a polyhedron shape, and the mean particle size is 44.2 nm. Scale bar, 100 nm. (c) TEM image of the silver nanoparticles after curing. The nanoparticles become sphere-shaped (dispersed with ethanol). Scale bar, 100 nm. (d) Microscopic image of the printed cathode ink on the surface of spin-coated P-PPV. The ink aggregates to form isolated islands. Scale bar, 400 μm. (e) Microscopic image of the silver ink on the surface of spin-coated PFNR2. The ink forms a continuous film. Scale bar, 400 μm. (f)J–V–Lcharacteristics of the devices. The solid markers representJdata, whereas the empty markers representLvalues. (g) LE–Jcharacteristics of the devices. Black for device A (ITO/PEDOT/P-PPV/Ba/Al), red for device B (ITO/PEDOT/P-PPV/PFNR2/Al), orange for device C (ITO/PEDOT/P-PPV/PFNR2/Ag), green for device D (ITO/PEDOT/P-PPV/PFNR2/nano Ag (ink-jetted)) and blue for device E (ITO/PEDOT/P-PPV/BL/nano Ag(ink-jetted). Figure 2: Single PLED device structure and performance with various EIL or BL and cathode combinations. ( a ) Device structure of the all-solution processed PLED single device with the printed nanoparticle cathode. ( b ) TEM image of the silver nanoparticles before curing. The nanoparticles have a polyhedron shape, and the mean particle size is 44.2 nm. Scale bar, 100 nm. ( c ) TEM image of the silver nanoparticles after curing. The nanoparticles become sphere-shaped (dispersed with ethanol). Scale bar, 100 nm. ( d ) Microscopic image of the printed cathode ink on the surface of spin-coated P-PPV. The ink aggregates to form isolated islands. Scale bar, 400 μm. ( e ) Microscopic image of the silver ink on the surface of spin-coated PFNR 2 . The ink forms a continuous film. Scale bar, 400 μm. ( f ) J–V–L characteristics of the devices. The solid markers represent J data, whereas the empty markers represent L values. ( g ) LE– J characteristics of the devices. Black for device A (ITO/PEDOT/P-PPV/Ba/Al), red for device B (ITO/PEDOT/P-PPV/PFNR 2 /Al), orange for device C (ITO/PEDOT/P-PPV/PFNR 2 /Ag), green for device D (ITO/PEDOT/P-PPV/PFNR 2 /nano Ag (ink-jetted)) and blue for device E (ITO/PEDOT/P-PPV/BL/nano Ag(ink-jetted). Full size image To form a uniform cathode film, the affinity of the cathode ink for the underlying organic layer is crucial. Figure 2d shows the annealed nano silver cathode on top of P-PPV. Because the nano silver ink with a polar solvent (triethylene glycol monoethyl ether) could not wet the non-polar P-PPV surface (the contact angle is 40.5°), the silver cathode formed isolated islands after annealing. In contrast, a uniform cathode layer was formed by the nano silver ink on the polar BL surface, as demonstrated in Fig. 2e , due to the wettability of the ink on the surface (the contact angle is 22°). To investigate the effects of the BL on PLED device performance, we fabricated five devices with different EIL (or BL) and cathode combinations using the same ITO/PEDOT/P-PPV layers: (A) a control device with a Ba/Al cathode and no EIL or BL; (B) spin-coated PFNR 2 with an evaporated Al cathode; (C) spin-coated PFNR 2 with an evaporated Ag cathode; (D) spin-coated PFNR 2 with an ink-jetted nano Ag cathode; and (E) spin-coated BL with an ink-jetted nano Ag cathode. The device fabrication is detailed in the Methods. Table 1 summarizes the performance of the five devices. The reflectances of the various Ag cathodes are indicated in Supplementary Fig. S1 . Unlike the specular reflection from the evaporated Ag cathode, the ink-jetted Ag cathode offers diffusive reflection. As illustrated in the emission spectra ( Supplementary Fig. S2 ), the additional PFNR 2 film broadened the emission spectrum in the long wavelength region due to the micro-cavity effect. Replacing the thin PFNR 2 film with the thick BL layer further extended the spectrum into the red region. The external quantum efficiencies (EQEs) of the devices were measured at a luminance ( L ) of 1,000 cd m −2 inside an integrating sphere, which accounted for the difference in the cathode reflectivity and the emission spectrum. Table 1 Performance of PLED devices with various EIL (or BL) and cathode combinations. Full size table As expected, control device A exhibits the best performance in terms of turn-on voltage ( V on ), L , luminous efficiency (LE) and EQE. When the low-work-function metal Ba was replaced by a PFNR 2 EIL (device B), the turn-on voltage increased by 1 V, the maximum L ( L max ) decreased by 52% and the maximum LE (LE max ) decreased by 32%. Replacing the evaporated Al cathode with evaporated Ag (device C) further reduced the device performance, because Ag has a higher work function than Al. When the ink-jetted nano silver ink served as the cathode, the performance of device D declined significantly with the worst performance among all the devices. However, upon substituting the PFNR 2 EIL with a BL, the performance of device E recovered to such a level that it exceeded that of device C with the evaporated Ag cathode. Upon examining the current density ( J )–voltage ( V )– L ) characteristics of the devices ( Fig. 2f ), we observe that the poor performance of device D is rooted in the leakage current caused by the penetration of the solvent into the emission layer. At the bias of −3 V, the current density of device D is 9.1 × 10 −3 mA cm −2 , one order of magnitude larger than that of device E with the BL at 5.4 × 10 −4 mA cm −2 . The J–V curve of device E is almost identical to that of device B, suggesting efficient electron injection from the ink-jetted nano Ag ink through the BL into the emission layer. In the plots of the LE ( Fig. 2g ), device E exhibits a typical dependence on the current density with the same trend as the devices with evaporated cathodes. The LE of device E reaches its maximum at low current density and then gradually declines as the current density increases. The reduced LE at high current density is attributed to the dissociation of the excitons by the excessive holes [28] . In contrast, device D without a BL exhibits a distinctly different trend, in which the LE monotonically increases. The monotonic increase of LE indicates that charge balance inside the emission layer of device D is not reached at the current density measured. Display A PLED display is a matrix of pixels, in which each pixel could be viewed as a miniature single PLED device. Under the driving of external chips, the pixels flash ‘row-by-row’ to produce a dynamic video. 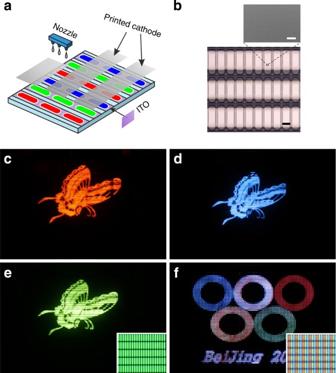Figure 3: Illustration of the display structure and photographs of monochrome and full-colour PLED displays. (a) Schematic illustration of the display structure of the full-colour display. (b) A microscopic image of the display’s backside. Scale bar, 100 μm. The inset is a SEM image of the silver nanoparticle cathode after curing,. Scale bar, 100 nm.(c) Red, (d) blue and (e) green monochrome displays. The inset of the green monochrome display is a microscopic image of the pixels under ultraviolet irradiation. (f) Full-color display with a microscopic image of the pixels under ultraviolet irradiation. Figure 3a presents the display structure and a microscopic image of the display. Table 2 lists the specifications of our 1.5-inch displays, which were fabricated using the all-solution process. To fabricate a monochrome display, the PEDOT:PSS hole-injection layer, the emission layer and the epoxy:PFNR 2 BL were sequentially deposited via spin-coating. To cure the BL, ultraviolet exposure followed by low-temperature (65 °C) annealing was applied. The light-emitting materials for the red, green and blue monochrome displays were MEH-PPV, P-PPV and G0 (ref. 29 ; Fig. 1 ), respectively. To improve the efficiency of the blue display, an additional hole-transport layer of poly( N -vinylcarbazole) was spin-casted on top of PEDOT:PSS before the deposition of G0. The respective single devices fabricated from different colour emitters exhibited consistent results compared with the representative green P-PPV single device described in the previous section. To fabricate a full-colour display, following the PEDOT:PSS blanket deposition, the blue emission layer of poly[3,7-dibenzothiophene-S,S-dioxide-co(9,9-dioctyl)-2,7-fluorene] (PF-FSO; Fig. 1 ) [30] was spin-coated. The common blue layer serves both as a receiving layer to reduce the leaking current and as a host layer to realize energy transfer in the red and green sub-pixels [31] , [32] . The red (PFO-DHTBT:P-PPV; ref. 33 ; Fig. 1 ), green (P-PPV) and blue (PF-FSO) polymer solutions were ink-jetted into the respective red, green and blue sub-pixels on top of the common blue layer to pattern the colours. The subsequent BL was processed similar to those in the monochrome displays. Figure 3: Illustration of the display structure and photographs of monochrome and full-colour PLED displays. ( a ) Schematic illustration of the display structure of the full-colour display. ( b ) A microscopic image of the display’s backside. Scale bar, 100 μm. The inset is a SEM image of the silver nanoparticle cathode after curing,. Scale bar, 100 nm. ( c ) Red, ( d ) blue and ( e ) green monochrome displays. The inset of the green monochrome display is a microscopic image of the pixels under ultraviolet irradiation. ( f ) Full-color display with a microscopic image of the pixels under ultraviolet irradiation. Full size image Table 2 Specifications of 1.5-inch (diagonal) all-solution processed PLED displays. Full size table The display cathodes were completed by ink-jetting the silver nanoparticle ink on top of the BL to form 64 parallel 0.28-mm wide rows, as illustrated in Fig. 3b . Because the overlapping area between the cathode rows and the ITO columns determines the actual aperture ratio of the pixels, it is desirable that the cathode rows be as wide as possible as long as the adjacent rows do not get short. After printing the cathode in air at room temperature, the panel was baked at 80 °C in nitrogen to remove the ink solvent. Because of the high flowability of the ink, high baking temperatures would distort and ruin the cathode line patterns. Following removal of the solvent, the panel was further baked at 140 °C for 30 min to sinter the silver nanoparticles and enable conductivity of the cathode lines. As illustrated in Fig. 3b , the cathode lines become solid and form a well-defined pattern without any defects after annealing. The scanning electron microscopy (SEM) image (the inset in Fig. 3b ) demonstrates that the sintered silver nanoparticles form a continuous and smooth film. To finalize the display, the panel was encapsulated with a glass cap with getters inside and bonded to the driver chips (SSD1332T1R1 from Solomon Systech Ltd.) controlled by the periphery circuits designed in our laboratory. Photographs of the monochrome and full-colour all-solution processed PLED displays are presented in Fig. 3c–f . The displays do not contain dead pixels or dead lines. The multifunctional BL provides protection for the organic functional layers, compatibility between the metal and the organic material, and electron injection from the metal to the organic material. The BL film formability and electron-injection ability were carefully investigated by varying the concentration of PFNR 2 in the epoxy (EP). As demonstrated in Fig. 4 , the film quality of the spin-coated BL films significantly improves as the doping concentration of PFNR 2 increases. Without any PFNR 2 , the pure epoxy cannot form a continuous film. A network of epoxy dot lines is clearly observed under the microscope. After a small amount of PFNR 2 is added to the epoxy (EP:PFNR 2 =10:0.05), a solid film can be formed; however, the film still contains many large epoxy clusters with surrounding cracks. When the weight ratio reaches EP:PFNR 2 =10:0.1, the epoxy clusters begin to shrink and disappear. The best film quality is achieved for the BL with EP:PFNR 2 =10:2. The electron-injection ability of the BL is characterized in the device structure of ITO/PEDOT/P-PPV/BL/Al. Table 3 summarizes the device performance, and Fig. 5a illustrate the J–V–L characteristics and the dependence of LE on the current density. 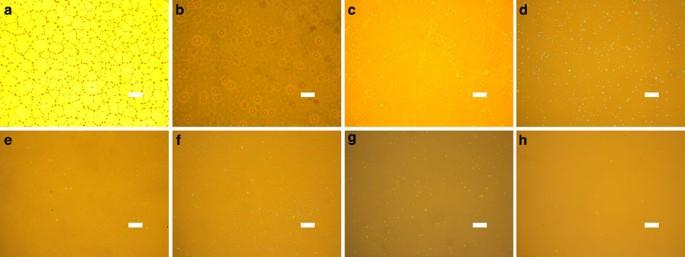Figure 4: Microscopic images of the BL films with various weight ratios. The weight ratios of EP:PFNR2are (a) 10:0, (b) 10:0.05, (c) 10:0.1, (d) 10:0.2, (e) 10:0.3, (f) 10:0.4, (g) 10:1 and (h) 10:2. Scale bars, 10 μm. Figure 4: Microscopic images of the BL films with various weight ratios. The weight ratios of EP:PFNR 2 are ( a ) 10:0, ( b ) 10:0.05, ( c ) 10:0.1, ( d ) 10:0.2, ( e ) 10:0.3, ( f ) 10:0.4, ( g ) 10:1 and ( h ) 10:2. Scale bars, 10 μm. Full size image Table 3 Performance of PLED devices with various BLs. 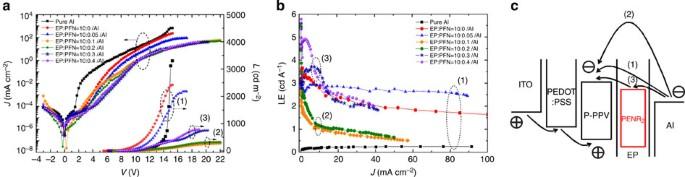Figure 5: Performance of PLED devices and proposed electron-injection mechanisms. (a)J–V–Lcharacteristics of the devices. (b) LE–Jcharacteristics of the devices. The weight ratios of BL range from 10:0 to 10:0.4. (c) Three electron-injection mechanisms. Path 1: the electrons are injected to the emitting layer through the BL cracks. The BL solvent facilitates the electron injection. Path 2: the percolation path through the BL is not established. The electrons must overcome the large injection barrier presented by the BL. Path 3: the percolation path of PFNR2in BL facilitates electron injection. Full size table Figure 5: Performance of PLED devices and proposed electron-injection mechanisms. ( a ) J–V – L characteristics of the devices. ( b ) LE– J characteristics of the devices. The weight ratios of BL range from 10:0 to 10:0.4. ( c ) Three electron-injection mechanisms. Path 1: the electrons are injected to the emitting layer through the BL cracks. The BL solvent facilitates the electron injection. Path 2: the percolation path through the BL is not established. The electrons must overcome the large injection barrier presented by the BL. Path 3: the percolation path of PFNR 2 in BL facilitates electron injection. Full size image Based on device performance, we can divide the devices into three groups. In the first group, which includes devices with EP:PFNR 2 =10:0 and 10:0.05, the device performances are similar to that of the Al cathode device without any BL. Because the BL cannot form a continuous film on top of the emission layer at an extremely low-doping concentration of PFNR 2 , direct contact is established between the aluminium cathode and the emission layer. Therefore, the electrons are injected through the P-PPV/Al interface instead of the insulating BL, as schematically illustrated by path (1) in Fig. 5c . In addition, the devices with low-doping concentrations of PFNR 2 exhibit better performance than the Al cathode device without any BL in terms of the LE. We attribute the efficiency improvement to the solvent methanol, which modifies the interface between the emission layer (P-PPV) and the cathode (Al) [34] . In the second group, which includes devices with EP:PFNR 2 =10:0.1 and 10:0.2, the device performances significantly decline. At the PFNR 2 -doping concentrations of 10:0.1 and 10:0.2, while the BL forms a continuous film without any cracks, the amount of PFNR 2 is too low to create a percolation path to help inject electrons. The electrons from the Al cathode must overcome the high potential barrier of the insulating BL to enter the emission layer, as path (2) in Fig. 5c illustrates. In the third group, which includes devices with EP:PFNR 2 =10:0.3 and 10:0.4, the device performances begin to recover, as illustrated in Fig. 5a . At the doping concentration of EP:PFNR 2 =10:0.3, the electrons could be efficiently injected into the emission layer, indicating the formation of percolation paths by PFNR 2 . The electron injection will follow path (3), as shown in Fig. 5c . As the PFNR 2 -doping concentration continues to increase, the device performance continues to improve until the doping concentration reaches 10:2. Further increasing the amount of PFNR 2 will damage the organic-layer-protecting function of the BL, reducing the device performance. Throughout our experiments, we selected the optimized doping concentration of EP:PFNR 2 =10:2. At the current stage, even with the optimized BL, the performance of the device with the ink-jetted nano Ag cathode is still inferior to that of the device with the evaporated Ba/Al cathode in terms of the EQE and operation voltage. The stabilities of the devices were investigated by stressing both the ink-jetted nano Ag cathode device and the evaporated Ag device ( Supplementary Fig. S3 ). Because of the limitations of our laboratory (lack of high-quality materials and industrial-grade clean room), neither device exhibits a long lifetime, with the device possessing the ink-jetted nano-silver cathode exhibiting a much shorter lifetime. In comparison, the light-emitting electrochemical cell device fabricated via Add-Vision Inc.’s fully solution process achieved a lifetime comparable to that of the PLED with the evaporated cathode. Because most damage to the ink-jetted nano Ag cathode device is caused by solvent permeation, by exploring different epoxies for BL and designing crosslinkable EILs, the lifetime of the device with the ink-jetted cathode would be improved to be on par with that of the devices with evaporated cathodes. Manufacturing organic flat panel displays without any vacuum or high-temperature processes promises a simple and cost-effective route towards inexpensive display technology, which would greatly have an impact on the industrial and electronic markets. The development of the all-solution processed display has answered three challenges encountered by the solution-based semiconductor industry: the development of solution-processed semiconductor devices (spin-coated and/or ink-jetted organic function layers in the display); the development of solution-processed interconnects (ink-jetted metal cathode lines); and the integration of organic functional components with inorganic functional components. In our approach, using a nano-sized silver-particle-based cathode ink instead of a micro-particle silver paste enables the cathodes to be inkjet printed to form fine patterns and reduces the risk of organic layers being pierced by micro-sized metal particles. The PFNR 2 -doped epoxy BL between the organic emission layer and the inorganic cathode layer not only protects the organics from the inorganics but also retains the necessary electron-injection functions. The solutions to these challenges pave the way towards the industrial roll-to-roll manufacturing of OLEDs. Materials and characterization methods All the chemicals and materials were purchased and used as received unless otherwise noted. PEDOT:PSS (Clevios P Al4083) was purchased from H. C. Starck GmbH, poly( N -vinylcarbazole) was purchased from Aldrich, and MEH-PPV and P-PPV were purchased from Canton OLedking Optoelectric Materials Co., Ltd. The other materials were synthesized in our laboratory. The film thicknesses were determined using a profilometer (Veeco Dektak 150). The surface resistance measurements were conducted using a four-point probe electrical measurement station (KDY-1 from Guangzhou Kunde Technology Co., Ltd.). SEM was performed on a Hitachi S-3700 SEM operated at 15 kV, and TEM was performed on a Hitachi H-7650 TEM operated at 80 kV. The J–L–V characteristics were measured using a Keithley 236 source-meter unit and a calibrated photodiode. The luminance was calibrated using a Photo Research PR-705 SpectraScan Spectrophotometer. PFNR 2 and the epoxy adhesive (ELC 2500CL) were dissolved into methanol at concentrations of 10 mg ml −1 and 100 mg ml −1 , respectively. A few drops of acetic acid were added into the PFNR 2 solution to improve solubility. The solutions of PFNR 2 and epoxy were mixed at the calculated volume ratios to form combined BLs with the desired weight ratios. Single device fabrication The ITO substrates (from the China Southern Glass Holding Corp.) were ultrasonically cleaned in sequence with acetone, detergent, deionized water and isopropyl alcohol. After ultraviolet ozone plasma treatment, the substrates were spin-coated with 50-nm thick PEDOT:PSS, followed by 10 min annealing at 200 °C inside a nitrogen-filled glove box (Vacuum Atmosphere Company). Next, 80 nm P-PPV layers were spin-coated on top of the PEDOT:PSS layer, followed by BL spin-coating. The BLs were cured in a ultraviolet curing chamber (ELC500 from Electro-Lite Corp., output 30 mW cm −2 ) for 2 min followed by annealing at 65 °C for 30 min. To prepare the cathode ink, 2 ml nano silver ink (DGP 40LT-15C) was filtered through a 0.45-μm hydrophobic filter and loaded into the cartridge of the inkjet printer (DMP 2831). Then, 1.9-mm wide rectangular ink patterns were printed on the devices with nozzle height of 1 mm and drop spacing of 25 μm. The effective light-emitting areas (1.9 × 7.5 mm 2 ) were defined by the overlap of the ITO anode and the silver nanoparticles cathode. After printing, the devices were baked at 80 °C in the nitrogen-filled glove box to remove the ink solvent. To improve the electrical conductivity of the cathodes, we re-printed the same patterns on the dried silver nanoparticle films. The typical thickness of the double-printed cathode was approximately 1 μm. After printing and drying, the devices were baked at 140 °C for 30 min to sinter the silver nanoparticles and enable conductivity of the cathodes. To fabricate the devices listed in Table 1 , on top of the P-PPV layer, we performed the following steps. Device A (ITO/PEDOT/P-PPV/Ba/Al): a 4-nm barium layer and a 200-nm aluminium layer were thermally evaporated as the cathode. Device B (ITO/PEDOT/P-PPV/PFNR 2 /Al): a 20-nm PFNR 2 layer was spin-coated, and a 200-nm aluminium layer was thermally evaporated as the cathode. Device C (ITO/PEDOT/P-PPV/PFNR 2 /Ag): a 20-nm PFNR 2 layer was spin-coated, and a 200-nm silver layer was thermally evaporated as the cathode. Device D (ITO/PEDOT/P-PPV/PFNR 2 / nano Ag(ink-jetted)): a 20-nm PFNR 2 layer was spin-coated, and the ink-jetted nano silver cathode was patterned and cured as described above. Device E (ITO/PEDOT/P-PPV/BL/nano Ag (ink-jetted)): a 50-nm BL was spin-coated, and the ink-jetted nano silver cathode was patterned and cured as described above. After the device structure and the fabrication process were optimized, all the experiments have been carried out for at least three times. How to cite this article: Zheng, H. et al. All-solution processed polymer light-emitting diode displays. Nat. Commun. 4:1971 doi: 10.1038/ncomms2971 (2013).